Bismuth atom tailoring of indium oxide surface frustrated Lewis pairs boosts heterogeneous CO2photocatalytic hydrogenation The surface frustrated Lewis pairs (SFLPs) on defect-laden metal oxides provide catalytic sites to activate H 2 and CO 2 molecules and enable efficient gas-phase CO 2 photocatalysis. Lattice engineering of metal oxides provides a useful strategy to tailor the reactivity of SFLPs. Herein, a one-step solvothermal synthesis is developed that enables isomorphic replacement of Lewis acidic site In 3+ ions in In 2 O 3 by single-site Bi 3+ ions, thereby enhancing the propensity to activate CO 2 molecules. The so-formed Bi x In 2-x O 3 materials prove to be three orders of magnitude more photoactive for the reverse water gas shift reaction than In 2 O 3 itself, while also exhibiting notable photoactivity towards methanol production. The increased solar absorption efficiency and efficient charge-separation and transfer of Bi x In 2-x O 3 also contribute to the improved photocatalytic performance. These traits exemplify the opportunities that exist for atom-scale engineering in heterogeneous CO 2 photocatalysis, another step towards the vision of the solar CO 2 refinery. The increasing energy demands of civil society have accelerated the consumption of coal, oil and natural gas, and associated greenhouse gas emissions. This situation is tipping the delicate balance of CO 2 in our atmosphere, leading to global warming. To this end, the photocatalytic hydrogenation of CO 2 into value-added chemicals and fuels has attracted global attention, touted a promising means of achieving a carbon-neutral economy [1] , [2] , [3] . Although materials such as Pd/Nb 2 O 5 [4] , Ru/Al 2 O 3 [5] , LDH nanosheets [6] , and Co-PS@SiO 2 [7] have been successfully employed as photocatalysts for CO 2 hydrogenation, a photocatalyst does not currently exist that can meet all the stringent requirements for practical application, including a broad solar response, high conversion efficiency, robust stability and low cost. This renders the design of a practical photocatalyst for CO 2 hydrogenation a challenge. Besides catalyst modifications designed to broaden spectral response and improve charge transfer efficiency, it is also important to accelerate conversion rates of H 2 or CO 2 on specially designed surface sites to boost photon and energy efficiency. Recently, surface frustrated Lewis pairs (SFLPs) have shown a propensity towards H 2 dissociation and CO 2 activation, a key enabler for many catalytic reactions, including hydrogenation, hydroamination and CO 2 reduction [8] , [9] , [10] . Generally speaking, SFLPs comprise proximal Lewis acidic and Lewis basic sites providing synergetic activation of reactant molecules. For example, SFLPs sites in the In 2 O 3– x (OH) y photocatalyst, comprises a coordinately unsaturated Lewis acidic In atom, proximal to an oxygen vacancy and an adjacent Lewis basic hydroxide group, enable the heterolysis of H 2 and reaction with CO 2 to form either CO or CH 3 OH [11] , [12] , [13] . As well, SFLPs involving coordinately unsaturated surface cobalt sites adjacent to surface hydroxides in the CoGeO 2 (OH) 2 photocatalyst form CH 4 from H 2 O and CO 2 [14] . In addition, SFLPs in oxygen vacancy laden CeO 2 bearing SFLPs catalyze the hydrogenation of alkenes and alkynes [15] . All of these cases utilize oxygen vacancies and hydroxides to engineer the catalytic activity of SFLPs. How to tailor the reactivity of the SFLPs themselves is rarely mentioned. Indium sesquioxide (In 2 O 3 ) is proving to be a promising catalyst for the thermal hydrogenation of CO 2 to CH 3 OH or CO [16] , [17] , [18] . Experimental and computational studies of CO 2 hydrogenation over oxygen vacancy laden In 2 O 3 revealed that methanol formation was favored over the reverse water gas shift (RWGS) reaction [19] , [20] . Methanol production was remarkably enhanced when In 2 O 3 was supported on ZrO 2 arising from electronic support effects [21] . A bifunctional catalyst composed of partially reduced In 2 O 3 supported on HZSM-5 could convert CO 2 directly into gasoline-range hydrocarbons with a 78.6% selectivity due to the synergistic effects of these two components [22] . By controlling the degree of non-stoichiometry in In 2 O 3– x , a black indium oxide catalyst, which utilized the entire solar spectrum, facilitated the photothermal RWGS reaction under ambient conditions with 100% selectivity [23] . Tailoring the electronic properties of In 2 O 3 can also be achieved via replacement of an indium atom in the lattice with a H 2 spillover palladium atom, although the rarity and cost of palladium could prove an issue for its practical implementation [24] . Bismuth, regarded as a “green” element, has a long and fascinating history [25] . The Incas in sixteenth century South America, made corrosion resistant bronzes for their knives by mixing bismuth with tin [26] . Paracelsus in fifteenth century Germany, recognized bismuth as a non-toxic brother to lead [27] . Since, it is finding myriad eco-friendly uses from cosmetics and personal care products to medicine and lubricants. Most recently it has proved to be a serious contender for replacing toxic lead halide perovskite materials in solar cells with non-toxic bismuth oxyiodide, retaining a comparable energy conversion efficiency of 22% [28] . Contextually, bismuth materials with layered structures and visible light absorption properties, exemplified by BiOX (X=Cl, Br, I), Bi 2 MO 6 (M=Mo, W), BiVO 4 and Bi 2 S 3 , behave as photocatalysts to be applied in dye degradation, water and carbon dioxide reduction [29] . Described herein, we developed a facile solvothermal route to achieve atom-precise substitution of Bi 3+ for In 3+ sites in In 2 O 3 and realize the tailor of the reactivity of SFLPs, as well as the electronic properties of In 2 O 3 . To amplify, by substituting cheaper and safer bismuth for indium in UV absorbing In 2 O 3 , one can create the broad-spectrum UV–Vis light absorber Bi x In 2– x O 3 . Significantly, single-site Bi 3+ substitution for In 3+ provides strong Lewis acidic/basic Bi 3+ –O 2− pairs that enhance CO 2 adsorption and activation, while Bi 6s 2 lone-pair electrons create mid-gap energy states. Atom-precise lattice engineering of this kind, boosts the reactivity of SFLPs and the harvesting efficiency of solar photons by Bi x In 2– x O 3 compared to In 2 O 3 , which enables 1000 times photoactivity enhancement of the RWGS reaction together with a noticeable increase in the production of solar methanol. Structural characterizations of single-site Bi x In 2– x O 3 Bi x In 2– x O 3 nanocrystals were prepared via a one-step solvothermal route, in which the molar ratio of Bi could be controlled by adjusting the concentration of Bi(NO 3 ) 3 and In(NO 3 ) 3 precursors. 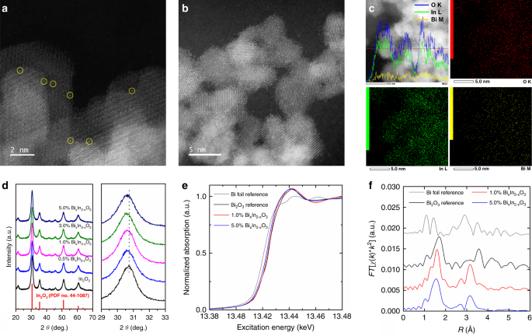Fig. 1: Structural characterizations of single-site Bi3+substituted BixIn2–xO3. aAberration-corrected STEM image of 1.0% BixIn2–xO3nanocrystals.bAberration-corrected STEM image of 5.0% BixIn2–xO3nanocrystals.cEDS mapping profiles of 5.0% BixIn2–xO3along the indicated red line.dPXRD patterns of BixIn2–xO3nanocrystals and pristine In2O3.eNormalized Bi L3-edge XANES spectra of 1.0% and 5.0% BixIn2–xO3, as well as Bi foil and Bi2O3references.fk3-Weighted Bi L3-edge Fourier-transform EXAFS spectra of 1.0% and 5.0% BixIn2–xO3,as well as Bi foil and Bi2O3references. The mole percent Bi content of each sample in the Bi x In 2– x O 3 series of nanocrystals was determined using inductively coupled plasma mass spectrometry (ICP-MS, Supplementary Table 1 ). Transmission electron microscopy (TEM) shows that the pristine In 2 O 3 nanocrystals are flower-like agglomerates of small nanocrystals with an average size of 3.7 nm (Supplementary Fig. 1 ). Bi 3+ substitution results in similarly sized Bi x In 2– x O 3 nanocrystals (3.5 nm) that show lattice fringes with a spacing of 2.92 Å, corresponding to the (222) plane of bcc In 2 O 3 (Supplementary Fig. 2 ). The obtained selected area electron diffraction pattern shown no evidence of any metallic Bi or Bi 2 O 3 . Most significantly, spherical aberration-corrected scanning transmission electron microscopy (STEM) images provide an insightful and distinct result, in which atomically dispersed single-site Bi atoms are revealed under these high-resolution imaging conditions as bright dots (Fig. 1a, b ). Energy-dispersive X-ray spectroscopy (EDS) line scans and elemental mapping (Fig. 1c and Supplementary Fig. 3 ) provided further evidence for the homogeneous distribution of elemental Bi in these Bi x In 2– x O 3 nanocrystals. Fig. 1: Structural characterizations of single-site Bi 3+ substituted Bi x In 2– x O 3 . a Aberration-corrected STEM image of 1.0% Bi x In 2– x O 3 nanocrystals. b Aberration-corrected STEM image of 5.0% Bi x In 2– x O 3 nanocrystals. c EDS mapping profiles of 5.0% Bi x In 2– x O 3 along the indicated red line. d PXRD patterns of Bi x In 2– x O 3 nanocrystals and pristine In 2 O 3 . e Normalized Bi L 3 -edge XANES spectra of 1.0% and 5.0% Bi x In 2– x O 3 , as well as Bi foil and Bi 2 O 3 references. f k 3 -Weighted Bi L 3 -edge Fourier-transform EXAFS spectra of 1.0% and 5.0% Bi x In 2– x O 3, as well as Bi foil and Bi 2 O 3 references. Full size image The phase structure of the obtained Bi x In 2– x O 3 nanocrystals was studied by powder X-ray diffraction (PXRD, Fig. 1d ). All the Bi x In 2– x O 3 nanocrystals displayed nearly identical XRD patterns diagnostic of face-centered cubic In 2 O 3 except that the diffraction peaks were shifted to lower 2 θ values relative to those of pristine In 2 O 3 . This result indicates In 3+ were isomorphously substituted by Bi 3+ , which has a larger ionic radius than In 3+ (i.e., 0.96 Å versus 0.81 Å). This conclusion is supported by the In 3d peaks in the corresponding X-ray photoelectron spectroscopy (XPS) spectra (Supplementary Fig. 4a ), which exhibited a gradual positive energy shift for Bi x In 2– x O 3 nanocrystals relative to pure In 2 O 3 , that is attributed to the higher electronegativity of Bi 3+ compared to In 3+ . The spin–orbit coupled doublet of Bi 4f XPS peaks at 158.6 eV and 163.9 eV define the oxidation state of bismuth as Bi 3+ rather than Bi 0 (Supplementary Fig. 4b ), following the isomorphous substitution of In 3+ by Bi 3+ . The electron paramagnetic resonance (EPR) spectra of Bi x In 2– x O 3 nanocrystals at both room temperature and 77 K revealed the absence of paramagnetic species, thereby providing further evidence for the lack of Bi 0 (Supplementary Fig. 5 ). Possibly EPR for semiconductors with high populations of [O]v occupied by electrons either does not exist or the existence of electronically degenerate ground states with fast electron relaxation and line broadening creates EPR silence. Maybe also the [O]v are devoid of trapped electrons or are doubly filled and hence diamagnetic and EPR silent. Further studies, such as 4 probe Van Der Paaw electrical conductivity measurements, are necessary to fully elucidate the conduction electron model. Synchrotron radiation-based X-ray absorption spectroscopy (XAS) was further used to obtain information regarding the local structural environment of these distributed Bi sites. The Bi L 3 − edge X-ray absorption near-edge structure (XANES) spectra in Fig. 1e reveal visible similarities between the 1.0% and 5.0% Bi x In 2– x O 3 sample spectra and that of the Bi 2 O 3 reference. These similarities are to be expected, given that Bi atoms in both Bi 2 O 3 and Bi x In 2– x O 3 lattices are expected to be octahedrally coordinated by oxygen atoms, leading to similarities in their structural and electronic properties. The Fourier-transformed Bi L 3 -edge extended X-ray absorption fine structure (EXAFS) spectra are presented in Fig. 1f . The similar positions of the Bi–O peak positions suggest that these bonds lengths in the Bi x In 2– x O 3 samples are similar to those in the Bi 2 O 3 reference. In stark contrast, though, the observed Bi–M peaks appear at distinctly different positions in the Bi x In 2– x O 3 spectra, revealing a distinct structural difference relative to the Bi 2 O 3 reference. In order to more accurately quantify these differences in bond length and structure, the spectra were also fitted to extract key structural parameter values (Supplementary Fig. 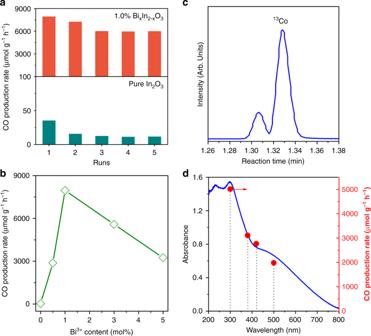Fig. 2: Photocatalytic performance in the batch reactor. aCO rate of pristine In2O3(down) and 1.0% BixIn2–xO3nanocrystals (up) in catalyzing hydrogenation of CO2under illumination.bCO rate as a function of Bi3+content for various BixIn2–xO3nanocrystals.cGC-MS plot of13CO produced from13CO2over 1.0% BixIn2–xO3nanocrystals.dCO rate as a function of absorption cutoff filter wavelength for 1.0% BixIn2–xO3nanocrystals. 6 and Supplementary Table 2 ). The resulting Bi–In bond lengths in the Bi x In 2– x O 3 samples are shorter than those found in the pristine Bi 2 O 3 lattice, though slightly longer than those observed in the pristine In 2 O 3 lattice. Relatively larger Debye-Waller coefficient values for the Bi–O peaks in Bi x In 2– x O 3 samples were also observed, reflecting a broader range of constituent Bi–O bond lengths. CO 2 hydrogenation performance The photocatalytic CO 2 hydrogenation activity of Bi x In 2– x O 3 nanocrystals was evaluated in a batch reactor under simulated solar light irradiation and using a 1:1 ratio of CO 2 and H 2 gases. In these experiments, the RWGS reaction (i.e., CO 2 + H 2 → CO + H 2 O) led to CO being the sole product detected. The CO production rates revealed that 1.0% Bi x In 2– x O 3 was more active than In 2 O 3 by approximately three orders of magnitude (Fig. 2a ), with an impressive peak rate of 8000 μmol g −1 h −1 for its first run, as compared to just 35 μmol g −1 h −1 for pristine In 2 O 3 . The estimated turnover frequency (TOF) of In 2 O 3 and 1.0% Bi x In 2– x O 3 is 0.42 h −1 and 93.6 h −1 , respectively ( Supplementary Note ), implying that substituting Bi atoms into In 2 O 3 nanocrystals significantly enhanced the photocatalytic activity towards CO 2 hydrogenation. Remarkably, this boost in catalytic activity was much more dramatic than that observed in analogous hydroxylated systems (i.e., Bi x In 2– x O 3 (OH) y ) [30] , thereby suggesting a distinct and potent mechanism of catalytic activity enhancement in Bi x In 2– x O 3 . 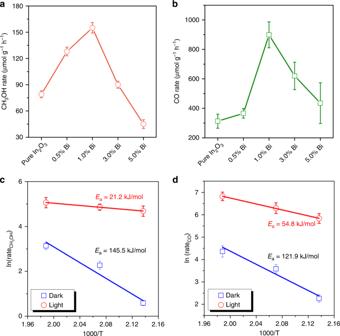Fig. 3: Catalytic performance in the flow reactor with and without light irradiation. aCH3OH production rates as a function of Bi3+content under light irradiation and at 230 °C.bCO production rates as a function of Bi3+content under light irradiation and at 230 °C.cArrhenius plots for CH3OH production rates of 1.0% BixIn2–xO3with and without solar irradiation.dArrhenius plots for CO production rates of 1.0% BixIn2–xO3with and without solar irradiation. Furthermore, such a CO production rate is much higher than some of the most active noble metal decorated photocatalysts (Supplementary Table 3 ). In addition, the 1.0% Bi x In 2– x O 3 was very stable, exhibiting a CO production rate that was still roughly 600 times greater than the 11 μmol g −1 h −1 exhibited by pristine In 2 O 3 under the same experimental conditions. In both cases, the CO production rate was observed to decrease over the course of five consecutive runs. Fig. 2: Photocatalytic performance in the batch reactor. a CO rate of pristine In 2 O 3 (down) and 1.0% Bi x In 2– x O 3 nanocrystals (up) in catalyzing hydrogenation of CO 2 under illumination. b CO rate as a function of Bi 3+ content for various Bi x In 2– x O 3 nanocrystals. c GC-MS plot of 13 CO produced from 13 CO 2 over 1.0% Bi x In 2– x O 3 nanocrystals. d CO rate as a function of absorption cutoff filter wavelength for 1.0% Bi x In 2– x O 3 nanocrystals. Full size image The actual bulk reaction temperature for In 2 O 3 and Bi x In 2– x O 3 tested by infrared camera is about 70 and 115 °C (Supplementary Fig. 7 ), respectively. The relatively low thermal energy supplied by solar light indicates the limited contribution of photothermal effect on the photocatalytic RWGS reaction. As an endothermic reaction, the rate of the RWGS is expected increase quite rapidly as a function of temperature. According to the Arrhenius Law, the rate should approximately double for every 10 °C increase in temperature. Thus, we would expect the reaction rate to increase by a factor of ~22.5, assuming that the bulk temperature of the catalyst accurately reflects the temperature of the catalytically active sites. Based on the rate of pristine In 2 O 3 (i.e., 35 μmol g −1 h −1 ), this would result in a rate increase to about 788 μmol  g −1 h −1 and account for about 10 % of the observed activity increase, thereby suggesting the existence of a significant photochemical effect. Notably, the marked increase in CO production rate upon substituting single-site Bi atoms into In 2 O 3 was highly dependent on the concentration of Bi atoms (Fig. 2b ). Meanwhile, isotopically labeled 13 CO 2 experiment confirmed that CO was the unequivocal product from photocatalytic CO 2 hydrogenation (Fig. 2c ). We also investigated the dependence of the CO production rate on the wavelength of light, to demonstrate the CO 2 hydrogenation proceeds mainly through a photocatalytic process. As seen in the action spectra shown in Fig. 2d and Supplementary Fig. 8 , the production rate of CO monotonically decreased with longer wavelengths of the light, which correlates with the optical absorption spectrum of pristine In 2 O 3 and Bi x In 2– x O 3 catalysts. It should also be mentioned that the CO production rate remained at about 2000 μmol g −1 h −1 on 1.0% Bi x In 2– x O 3 , even when a 500 nm cutoff filter was applied, thus implying that Bi x In 2– x O 3 nanocrystals can function as broadband, green photocatalysis for harvesting solar energy. In light of the promising performance of Bi x In 2– x O 3 nanocrystals towards gas-phase CO 2 hydrogenation, this new catalyst was also studied for solar methanol production in a flow reactor at 230 °C, both with and without light irradiation. As shown in Supplementary Fig. 9 , all catalysts exhibited similarly low CO and CH 3 OH production rates under purely thermal conditions; however, a remarkable enhancement in the production rates of CO and CH 3 OH was obtained on changing from dark to light conditions. In this case, pristine In 2 O 3 exhibited CO and CH 3 OH production rates of 312 and 82 μmol g −1 h −1 , respectively (Fig. 3a, b ). In comparison, the single-site Bi x In 2– x O 3 samples exhibited much better activities for both CO and CH 3 OH production, with 1.0% Bi x In 2– x O 3 exhibiting the highest CO and CH 3 OH production rates of 918 μmol g −1 h −1 and 158 μmol g −1 h −1 , respectively. Overall, the measured activities of the Bi x In 2– x O 3 samples were highly dependent on Bi content and showed a volcano-shaped trend. The volcano trend of the activity towards CO 2 hydrogenation versus the extent of In 3+ substitution by the larger, more electronegative, 6s 2 stereochemically active lone-pair containing Bi 3+ , can be attributed to a subtle interplay of numerous and competing intertwined properties: chemical effects (e.g., influence of surface Lewis acidity and basicity of In-O-In, In-O-Bi, Bi-O-Bi sites on CO 2 -H 2 adsorption, activation, reaction processes) and physical effects (e.g., photogenerated electron and hole charge-separation and charge-trapping by bismuth and oxygen vacancy mid-gap states). Fig. 3: Catalytic performance in the flow reactor with and without light irradiation. a CH 3 OH production rates as a function of Bi 3+ content under light irradiation and at 230 °C. b CO production rates as a function of Bi 3+ content under light irradiation and at 230 °C. c Arrhenius plots for CH 3 OH production rates of 1.0% Bi x In 2– x O 3 with and without solar irradiation. d Arrhenius plots for CO production rates of 1.0% Bi x In 2– x O 3 with and without solar irradiation. Full size image The CH 3 OH and CO production rates of Bi x In 2– x O 3 nanocrystals showed negligible deactivation, even after 50 h of continuous testing under light irradiation at 230 °C (Supplementary Fig. 10a ), suggesting their excellent catalytic stability. The recorded XRD patterns, TEM images and XPS spectra (Supplementary Fig. 10b–d ) for the spent Bi x In 2– x O 3 photocatalysts after 50 h of reaction demonstrate that, except for a slight increase in particle size, the phase and oxidation states of the nanocrystals were well maintained, confirming their favorable structural stability. To obtain more information on the origin of the activity enhancement under flow reaction conditions, activity tests were also conducted at lower reaction temperatures, beginning where products can be observed (130, 195, and 210 °C), with and without light irradiation (Supplementary Fig. 11 ). The drastic activity difference between dark and light conditions lend further support confirmed the contribution of the photochemical effect on CO and CH 3 OH production. Moreover, based on the Arrhenius plots for 1.0% Bi x In 2– x O 3 , the apparent activation energy for the CO and CH 3 OH photochemical processes are much lower than the thermochemical ones (Fig. 3c, d ), reflecting the solar advantage for the excited-state reaction pathway relative to the ground state pathway [31] . Photocatalytic reaction pathway The photocatalytic CO 2 hydrogenation reaction involves photon-absorption, electron-hole separation, and CO 2 adsorption/activation processes. The first two steps are closely related to the intrinsic nature of the photocatalyst, while the third is highly dependent on the gas-solid interface. A significant red shift occurs in the absorption edge of the UV–Vis spectra for all Bi x In 2– x O 3 samples (Fig. 4a ), along with an enhanced tail above 440 nm, which grows with Bi 3+ content and is accompanied by a change in color from cream to rust (Supplementary Fig. 12 ). This is consistent with the simulated band structures that show the introduction of Bi 3+ can leads to the formation of mid-gap states in the bandgap of In 2 O 3 (Fig. 4b, c ). The total density of states (DOS) and partial density of states (PDOS) (Supplementary Fig. 13 ) can further reveal that the substitution of Bi at the In site induces mid-gap energy states with Bi 6s states below the conduction band edge of In 2 O 3 and is consistent with the reported results in this paper [32] , [33] , [34] . Fig. 4: Electronic structures of Bi x In 2– x O 3 . a Diffuse reflectance spectra of pristine In 2 O 3 and various Bi x In 2– x O 3 nanocrystals. b The simulated band structure and DOS plots of pristine In 2 O 3 . c The simulated band structure and DOS plots of Bi x In 2– x O 3 nanocrystals. d Room-temperature PL spectra of pristine In 2 O 3 and 1.0% Bi x In 2– x O 3 nanocrystals using an excitation wavelength of 325 nm. e Schematic illustrating charge carrier recombination pathways on surface defects states (SFLPs) and enabling CO 2 hydrogenation reactions. Full size image To understand the photogenerated charge transfer mechanism, the room-temperature photoluminescence (PL) spectra of pristine In 2 O 3 and 1.0% Bi x In 2– x O 3 nanocrystals are shown in Fig. 4d . The pristine In 2 O 3 nanocrystals exhibited a strong green emission peak centered at ca. 440 nm, originating from the radiative recombination of photo-excited electrons trapped in mid-gap oxygen vacancy states with photogenerated holes in the valence band [35] . The existence of oxygen vacancies is further evidenced by the O 1 s core level XPS spectra (Supplementary Fig. 14 ). In contrast, the incorporation of single-site Bi into In 2 O 3 leads to weakening and broadening of the PL emission peak. This can be explained in two ways. One is that the substitutional Bi 3+ slightly decreases the concentration of oxygen vacancies (Supplementary Fig. 15 ), which would decrease the intensity due to electron-hole radiative recombination. Alternatively, the substituted Bi 3+ states lying below the conduction band of In 2 O 3 could also act as traps capturing photo-excited electrons and inhibiting electron-hole recombination emission, resulting in lower PL emission. Thus, as illustrated in Fig. 4e , the substituted Bi 3+ sites (denoted as Bi’), oxygen vacancies [O], coordinately unsaturated indium In’ sites and oxygen O’ sites, exist as mid-gap defect states (comprising surface frustrated Lewis pairs, SFLPs) in the bandgap of Bi x In 2– x O 3 , can function as traps for photogenerated electrons and holes enabling the reaction between CO 2 /H 2 [36] , [37] . This results in the quenching of steady-state PL emission as well as a slight shortening of the average fluorescence lifetime from 120 to 110 ps, probed by time-resolved PL spectroscopy (Supplementary Fig. 16 ). Albeit small, this reduction of the fluorescence lifetime, suggests that, relative to In 2 O 3 , single-site Bi atoms can increase the occurrence of competitive non-radiative relaxation processes in Bi x In 2– x O 3 [38] , [39] , [40] . Apart from its effect on the electronic structure and charge transfer, single-site Bi 3+ substitution is also expected to strengthen the adsorption-bonding-activating ability of Bi x In 2– x O 3 toward CO 2 . 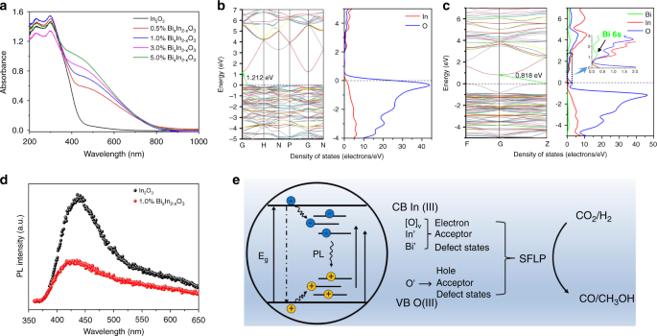Fig. 4: Electronic structures of BixIn2–xO3. aDiffuse reflectance spectra of pristine In2O3and various BixIn2–xO3nanocrystals.bThe simulated band structure and DOS plots of pristine In2O3.cThe simulated band structure and DOS plots of BixIn2–xO3nanocrystals.dRoom-temperature PL spectra of pristine In2O3and 1.0% BixIn2–xO3nanocrystals using an excitation wavelength of 325 nm.eSchematic illustrating charge carrier recombination pathways on surface defects states (SFLPs) and enabling CO2hydrogenation reactions. The textural structure of Bi x In 2– x O 3 including surface area, pore volume and pore size show obvious improvements and could favor the adsorption of CO 2 reactants (Supplementary Table 4 and Supplementary Fig. 17 ). With respect to the surface chemistry, CO 2 can bond through its carbon atom and oxygen atoms to either the surface oxygen atoms, metal sites, or directly with the oxygen vacancies of metal oxides (Supplementary Fig. 18 ) [41] , [42] , [43] . To investigate the effect of Bi 3+ substitution on the interaction between CO 2 and Bi x In 2– x O 3 or pristine In 2 O 3 nanocrystals, CO 2 temperature-programmed desorption (CO 2 -TPD) measurements were initially performed. As shown in Fig. 5a , one broad desorption peak at around 100 °C, corresponding to physically adsorbed CO 2 , is observed for all Bi x In 2– x O 3 nanocrystals and pristine In 2 O 3 . A significant desorption peak is clearly observed at 256 °C for pristine In 2 O 3 and can be attributed to the chemical desorption of CO 2 that is binding with oxygen vacancies to form bent CO 2 δ− species [44] . Since Bi 3+ substitution results in fewer oxygen vacancies, this peak intensity gradually decreases with increased Bi 3+ doping of Bi x In 2– x O 3 nanocrystals and shifts slightly to higher temperatures (as high as 275 °C for 5.0 % Bi x In 2– x O 3 ), implying that the binding strength of CO 2 and oxygen vacancies is remarkably enhanced. Moreover, weak desorption peaks at higher temperatures (300 to 600 °C) were clearly observed for In 2 O 3 , and can be assigned to the decomposition of surface HCO 3 − and CO 3 2− species [45] . After single-site Bi 3+ substitution, typical desorption peaks can also be clearly identified and show a slight shift to higher temperatures, again indicating that these surface species are binding more strongly to the surface. Fig. 5: In situ DRIFTS experiments of CO 2 adsorption and CO 2 hydrogenation. a CO 2 -TPD profiles. b In situ DRIFTS spectra for the adsorption of CO 2 on 1.0% Bi x In 2– x O 3 nanocrystals (up) and pure In 2 O 3 (down). c In situ DRIFTS spectra of surface species under reaction conditions on 1.0% Bi x In 2– x O 3 nanocrystals (up) and pure In 2 O 3 (down). Full size image In situ diffuse reflectance infrared Fourier-transform spectroscopy (DRIFTS) experiments were further carried out to identify surface species. 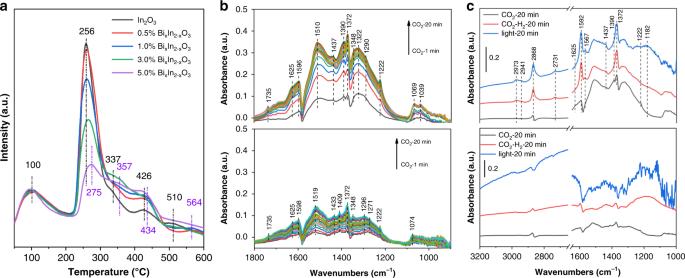Fig. 5: In situ DRIFTS experiments of CO2adsorption and CO2hydrogenation. aCO2-TPD profiles.bIn situ DRIFTS spectra for the adsorption of CO2on 1.0% BixIn2–xO3nanocrystals (up) and pure In2O3(down).cIn situ DRIFTS spectra of surface species under reaction conditions on 1.0% BixIn2–xO3nanocrystals (up) and pure In2O3(down). 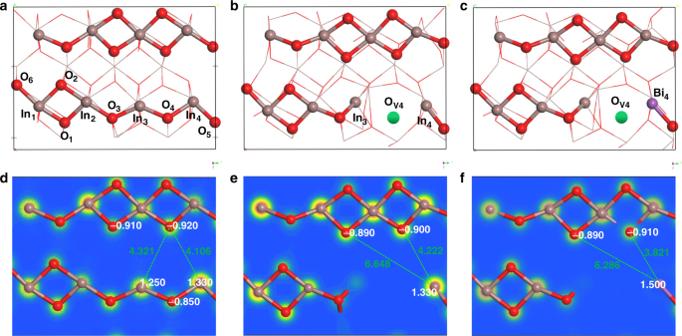Fig. 6: Schematic images of the reactivity of SFLPs in single-site Bi3+substituted BixIn2–xO3. aOptimized structure of perfect In2O3(110).bOptimized structure of defective In2O3(110) with one oxygen vacancy.cOptimized structure of BixIn2–xO3(110) with Bi3+substitution.dElectron-density isosurface of perfect In2O3(110).eElectron-density isosurface of defective In2O3(110) with one oxygen vacancy.fElectron-density isosurface of BixIn2–xO3(110) with Bi3+substitution. Figure 5b show the transient evolution of the surface species during CO 2 adsorption over 1.0% Bi x In 2– x O 3 nanocrystals. The bands at 1510 and 1372 cm −1 are assigned to the asymmetric and symmetric OCO stretching modes of monodentate carbonates ( m -CO 3 2− ). The features at 1549 and 1330 cm −1 are attributed to the asymmetric and symmetric OCO stretching modes of bidentate carbonates ( b -CO 3 2− ). The bent CO 2 δ− species adsorbed at oxygen vacancy sites can be identified by two bands at 1596 and 1348 cm −1 , corresponding to the asymmetric and symmetric stretching modes, respectively. The appearance of bands at 1625, 1437, 1390, and 1222 cm −1 indicates the formation of bicarbonate species (HCO 3 − ). Moreover, a small amount of a linearly adsorbed CO 2 species with bands appearing between 1000 and 1100 cm −1 can also be observed. Thus, via DRIFTS measurements, all the surface species observed during CO 2 -TPD measurements, CO 3 2− , HCO 3 − and CO 2 δ− , were observed and identified on Bi x In 2– x O 3 nanocrystals. All these surface species can be observed on pristine In 2 O 3 ; however, the peak intensities of these species are weaker than that on Bi x In 2– x O 3 nanocrystals, suggesting the improved CO 2 adsorption-bonding-activating capacity after Bi 3+ substitution. Density functional theory (DFT) slab calculations were further carried out to unravel the promotion effect of Bi 3+ substitution on In 2 O 3 . The perfect In 2 O 3 (110) surface was initially selected as it has proven to be most thermodynamically stable [20] , [46] . The defective In 2 O 3 (110) surface with an oxygen vacancy at the O 4 site was then created owing to the more favorable ability for CO 2 activation and hydrogenation [19] . Following then, we examined the possibility of Bi 3+ substitution at the In site. As shown in Fig. 6a , the perfect In 2 O 3 (110) surface consists of chains of In and O atoms, with the numbering In and O atoms along the chain as repeating unit. The surface In and O in the chain are adjacent and contiguous to each other, forming a classic Lewis acid-base adjunct, whereas the unbonded In 3 and In 4 in the chain and O in the top layer show a distance of 4.106 and 4.312 Å, respectively, which may deliver SFLPs-like activity (Fig. 6d ). However, the electronic interactions between In 3 or In 4 and its neighboring O 4 will block the function of In 3 -O or In 4 -O pairs. Therefore, the removal of oxygen atom at the O 4 site is the prerequisite to construct a pair of unbonded Lewis acid and base sites. When the O 4 atom is removed, two In atoms (In 3 and In 4 ) are coordinatively unsaturated and one oxygen vacancy (O V4 ) is produced (Fig. 6b ). However, in this case, only one In atom (In 4 ) locates at the surface while the other one (In 3 ) moves to the inner atomic layer. The surface In 4 atom is found to be surrounded by two adjacent oxygen atoms, of which the In 4 -O with a distance of 4.222 Å can construct a SFLPs site (Fig. 6e ). We further investigated the effect of Bi 3+ substitution at In 4 site on the configuration and charge population (Fig. 6c, f ). As compared to In 4 -O configuration, Bi 4 -O shows a shorter distance (3.821 Å) but can still fall in the domain of solid SFLPs. On the other hand, the Bader charge calculations show that the related Lewis acid Bi 3+ and Lewis base O 2− involve atomic local charges of +1.500 e and −0.910 e, respectively, which is higher than that of the In 3+ and O 2− pair (+1.300 e and −0.900 e). The larger charge difference between the Lewis acid and Lewis base pairs in the Bi x In 2– x O 3 compared with that of defective In 2 O 3 would form more active Lewis acid-base pairs than the In 2 O 3 pair can muster, and therefore could deliver a higher capability to activate CO 2 molecules, consistent well with the DRIFTs and CO 2 -TPD results. Fig. 6: Schematic images of the reactivity of SFLPs in single-site Bi 3+ substituted Bi x In 2 –x O 3 . a Optimized structure of perfect In 2 O 3 (110). b Optimized structure of defective In 2 O 3 (110) with one oxygen vacancy. c Optimized structure of Bi x In 2– x O 3 (110) with Bi 3+ substitution. d Electron-density isosurface of perfect In 2 O 3 (110). e Electron-density isosurface of defective In 2 O 3 (110) with one oxygen vacancy. f Electron-density isosurface of Bi x In 2– x O 3 (110) with Bi 3+ substitution. Full size image In the photo-excited state of a SFLPs system, the Lewis acidity and Lewis basicity have been shown to increase as compared with the ground state, thereby facilitating the photochemical CO 2 hydrogenation, with a decrease in activation energy. To get more insight into the improved activity from Bi 3+ substitution, in situ DRIFTS experiments were further performed under reaction conditions to detect the reaction intermediates and uncover the photocatalytic pathway in the CO 2 hydrogenation process. As shown in Fig. 5c , when the Bi x In 2– x O 3 nanocrystals were exposed to the mixture of CO 2 and H 2 gases, bidentate formate (*HCOO), methoxy (*H 3 CO) and carboxylate (*CO 2 ) [47] , were the three principal intermediates observed from the transformation of bicarbonate and carbonate species, as evidenced by the decrease and disappearance of characteristic bands at 1510, 1390, and 1222 cm −1 . The *HCOO species can be linked to fingerprint modes at 2973 and 2731 cm −1 , which correspond to a combination of the CH bending and OCO stretching modes [47] , [48] . The bands at 1592 and 1370 cm −1 can be assigned to the asymmetric and symmetric OCO stretching modes while that at 2868 cm −1 is attributed to the CH stretching mode of the same species [47] , [49] , [50] . The *H 3 CO species is signaled by diagnostic modes at 2941 and 2838 cm −1 that are assigned to the CH 3 stretching modes and the band at 1182 cm −1 is attributed to the CO stretching mode of bridged methoxide species [47] , [48] , [51] . In addition to *HCOO and *H 3 CO, *CO 2 species were also observed, with bands at 1567 and 1379 cm −1 that can be associated with the OCO stretching modes. Under light irradiation, all intermediates showed an increase in band intensity (Supplementary Fig. 19 ), thereby confirming the photochemical effect of CO 2 hydrogenation, and is consistent with the activity results. From these DRIFT results, CO 2 hydrogenation over Bi x In 2– x O 3 may proceed via two major reaction pathways featured by both formate intermediate and CO intermediate, which has been well established for the In 2 O 3- x (OH) y systems [12] . In the case of pristine In 2 O 3 (Fig. 5c and Supplementary Fig. 20 ), *HCOO and *H 3 CO species of virtually insignificant intensity were observed for CO 2 hydrogenation, and light irradiation resulted in much noisier peaks. This further indicates the moderate catalytic performance of pristine In 2 O 3 and the significant promotion effect resulting from single-site Bi 3+ substitution. To corroborate these experimental observations, free energy profiles for CO 2 hydrogenation via the proposed RWGS pathway over Bi x In 2– x O 3 and pristine In 2 O 3 were calculated (Supplementary Fig. 21 ). It can be seen that the H 2 dissociation into H* on pristine In 2 O 3 (defective type with one oxygen vacancy) is the rate-limiting step and endothermic with an activation energy barrier of 1.47 eV. Importantly, compared with pristine In 2 O 3 , the Bi x In 2– x O 3 exhibits a negative Δ G value of −0.05 eV for the H 2 dissociation, which implies that the H 2 dissociation into H* on the surface of Bi x In 2– x O 3 is energetically favorable. This result indicates that the single-site Bi 3+ substituted nanostructure has more active Lewis acid-base pairs than the In 2 O 3 pair can muster, and therefore can strongly polarize H–H bonds and dissociate H 2 molecules into *H. The proceeding hydrogenation reactions of H* with CO 2 on the surface of In 2 O 3 and Bi x In 2– x O 3 are similar. However, benefiting from the favorable H 2 dissociation, Bi x In 2– x O 3 shows a much-lowered reaction energy profile for CO and H 2 O formation than pristine In 2 O 3 . In summary, we have demonstrated a one-step solvothermal route towards atom-precise isomorphic substitution of In 3+ in In 2 O 3 by Bi 3+ to generate Bi x In 2– x O 3 materials with broad-spectrum UV–Vis absorption. The incorporation of single-site Bi atoms in the In 2 O 3 host lattice provides strong Lewis acid-base Bi 3+ –O 2− pairs to enhance CO 2 adsorption and activation, resulting in distinctly enhanced reaction rates relative to those observed for pristine In 2 O 3 and other indium oxide-based catalysts. The Bi 6s 2 lone pairs create mid-gap energy states, which can increase the harvesting of solar photons and favor the generation and separation of photo-induced charge carriers. Remarkably, single-site Bi 3+ -substituted Bi x In 2– x O 3 proves to be a highly efficient and stable photocatalyst, achieving an impressive CO production rate three orders of magnitude greater than that of pristine In 2 O 3 , with notable photoactivity towards solar methanol. In addition to increased activity catalytic sites, the greening of indium oxide by single-site bismuth atom substitution represents a new approach to CO 2 photocatalyst engineering and is a further step towards the vision of a solar CO 2 refinery. Synthesis of In 2 O 3 and Bi x In 2– x O 3 Pristine In 2 O 3 nanocrystals were prepared via a simple solvothermal route. In a typical synthesis, 0.3 g of In(NO 3 ) 3 •4.5H 2 O was dissolved in 17 mL anhydrous dimethylformamide solution. After stirring for 30 min, the obtained homogeneous solution was transferred into a Teflon-lined stainless steel autoclave and then heated at 150 °C for 24 h. After being cooled to room temperature, the light-yellow product was collected through centrifugation, washed with ethanol and water, and finally dried at 60 °C in vacuum. Bi 3+ -substituted In 2 O 3 nanocrystals were prepared using the same method employed for pristine In 2 O 3 , except that various amounts of Bi(NO 3 ) 3 •5H 2 O were added to the indium solution prior to solvothermal reaction. Material characterizations The content of Bi in Bi x In 2– x O 3 was determined using an inductively coupled plasma mass spectroscopy (ICP-MS) instrument (Optima 7300 DV). Powder X-ray diffraction (PXRD) was performed on a Bruker D2-Phaser X-ray diffractometer, using Cu Kα radiation at 30 kV. X-ray photoelectron spectroscopy (XPS) was performed using a PerkinElmer Phi 5500 ESCA spectrometer in an ultrahigh vacuum chamber with a base pressure of 1 × 10 −9 Torr. The spectrometer used an Al Kα X-ray source operating at 15 kV and 27 mA. The samples were coated onto carbon tape prior to analysis and all results were calibrated to C1s 284.5 eV. EPR spectra were obtained at room temperature and 77 K using a Bruker A-300-EPR X-band spectrometer. Transmission electron microscopy (TEM) measurements were conducted using a JEM–2010 microscope working at 200 kV. The double spherical aberration-corrected scanning transmission electron microscope (STEM) images were obtained on an FEI Themis Z instrument. X-ray absorption spectra were collected at the BL14W beamline of the Shanghai Synchrotron Radiation Facility (SSRF). The storage ring of the SSRF was operated at 3.5 GeV with a stable current of 200 mA. Using a Si(111) double-crystal monochromator, the data collection was carried out in fluorescence mode using Lytle detector. All spectra were collected under ambient conditions. Diffuse reflectance spectra (DRS) of the powders were obtained for dry-pressed disk samples using a Cary 500 Scan Spectrophotometer (Varian, USA) over a range of 200 to 800 nm. Barium sulfate (BaSO 4 ) was used as a reflectance standard. Room-temperature photoluminescence (PL) spectra were measured on an FL/FS 920 (Edinburgh Instruments) system equipped with a 450 W Xe arc lamp as the excitation source and a red sensitive Peltier element-cooled Hamamatsu R2658 PMT as the detector. Time-resolved fluorescence decay spectra were recorded on the Delta Pro (HORIBA instruments) using a 357 nm laser as the excitation source. BET surface area analyses were performed on an ASAP2020 M apparatus (Micromeritics Instrument Corp., USA) with the samples degassing in vacuum at 110 °C for 10 h and then measuring at 77 K. The CO 2 temperature-programmed desorption (CO 2 -TPD) measurements were carried out on AutoChem II 2920 Version. The density functional theory (DFT) calculations were performed using the Cambridge Sequential Total Energy Package (CASTEP) computational codes. During the geometry optimization, lattice parameters and atomic positions were optimized simultaneously. Based on the experimental data, we replaced one In with Bi in the cell as the In 15 BiO 24 model and deleted one of the oxygen atom that were coordinating with Bi to establish one In 15 BiO 23 (O Vacancy ) model. For calculating the electronic structures and density of states, the geometry optimization of In 2 O 3 and In 15 BiO 23 (O Vacancy ) were calculated by the PBE method within Generalized Gradient-corrected Approximation (GGA), using the exchange-correlation potential. The Vanderbilt ultrasoft pseudopotential with a cutoff energy of 380 eV was used to ensure the precision of the results. Brillouin zone integration was represented using the K-point sampling scheme of 3 ×  3 × 3 Monkhorst–Pack scheme. The convergence tolerance for geometry optimization was selected with the differences in total energy (5.0 × 10 −6 eV/atom), the maximal ionic Hellmann–Feynman force (1.0 × 10 −2 eV Å −1 ), the stress tensor (2.0 × 10 −2 GPa), and the maximal displacement (5.0 × 10 −4 Å). Gas-phase CO 2 hydrogenation tests Batch reactions were conducted in a custom-built 1.5 mL stainless steel batch reactor with a fused-silica viewport sealed with Viton O-rings. The reactor with ∼ 4.5 mg of catalyst on a borosilicate film support was evacuated using an Alcatel dry pump prior to being purged with the reactant high-purity H 2 reactant gas. After purging the reactor, it was filled with a 1:1 stoichiometric mixture of H 2 (99.9995%) and CO 2 (99.999%) until the total pressure reached 30 psi. The reactor was irradiated with a 300 W Xe lamp for a duration of 1 h without external heating. Product gases were analyzed using flame ionization and thermal conductivity detectors installed in a SRI-8610 gas chromatograph equipped with 3 in. Mole Sieve 13a and 6 in. Haysep D column. Isotopically labeled tracing experiments were performed using 13 CO 2 (99.9 at%, Sigma-Aldrich). Isotope distributions in the product gases were measured using an Agilent 7890A gas chromatograph-mass spectrometer with a 60 m GS-carbon plot column, leading to the mass spectrometer. Flow experiments were carried out in a fixed-bed tubular reactor with ∼ 10 mg of catalyst material being packed into a quartz tube and immobilized at both ends with quartz wool. The quartz tube had an inner diameter of 2 mm with a wall thickness of 0.5 mm, and was placed into a groove carved out into a copper block. An OMEGA temperature controller was attached to two heating cartridges inserted into the copper block and a thermocouple was inserted into the quartz tube contacting the catalyst but covered by the quartz wool. A 300 W Xe arc lamp illuminated the catalyst plug at a measured intensity of 2 W cm −2 . CO 2 and H 2 were flowed through with a 1:3 ratio (1 sccm CO 2 , 3 sccm H 2 ). The amounts of CO and CH 3 OH produced were determined using gas chromatography-mass spectrometry (GC-MS, 7890B and 5977A, Agilent) using a He carrier gas. In situ DRIFT studies The in situ DRIFTS measurements were performed to detect the surface intermediates over pristine In 2 O 3 and Bi x In 2– x O 3 nanocrystals under reaction conditions. The spectra were collected using a Fourier-transform infrared spectroscopy spectrometer (Thermo, Nicolet 6700) equipped with an MCT detector. Before measurement, the catalyst was purged with He at 250 °C for 2 h. The catalyst was subsequently cooled down to 230 °C. The background spectrum with a resolution of 4 cm −1 was obtained at 230 °C in He flow. Then the catalyst was exposed to a mixture of CO 2 , H 2 , and He (1 sccm CO 2 , 3 sccm H 2 , and 16 sccm He, respectively) in dark and light conditions for different times. The in situ DRIFT spectra were recorded by collecting 32 scans at 4 cm −1 resolutions.